Visually induced initiation ofDrosophilainnate courtship-like following pursuit is mediated by central excitatory state The courtship ritual of male Drosophila represents an innate behaviour that is initiated by female-derived sensory stimuli. Here we report that moving light spots can induce courtship-like following pursuit in tethered wild-type male flies provided the fly is primed by optogenetic stimulation of specific dsx -expressing neuronal clusters in the lateral protocerebrum (LPR). Namely, stimulation of the pC1 neuronal cluster initiates unilateral wing extension and vibration of both sides, whereas stimulation of the pC2l cluster initiates only contralateral wing displays. In addition, stimulation of pC2l but not pC1 neurons induced abdominal bending and proboscis extension. Ca 2+ imaging of the pC1 cluster revealed periodic Ca 2+ rises, each corresponding to a turn of the male fly during courtship. In contrast, group-reared fru mutant males exhibit light spot-induced courtship pursuit without optogenetic priming. Ca 2+ imaging revealed enhanced responses of LPR neurons to visual stimuli in the mutants, suggesting a neural correlate of the light spot-induced courtship behaviour. D rosophila melanogaster males are highly sensitive to moving objects. Visual motion typically results in orienting and chasing behaviours, which are often accompanied by unilateral wing extension and vibration, two hallmarks of courtship behaviour [1] , [2] , [3] , [4] . However, such courtship-like behaviour quickly wanes unless the moving object is a female [1] , [2] , [3] , [4] . Using an actuated magnet as a dummy, Agrawal et al . [5] succeeded in inducing courtship pursuit in a freely moving male fly that persisted longer when the dummy was perfumed with a pheromone blend, that is, hexane extracts of cuticular hydrocarbons, from the body of a conspecific female. This observation suggests that the combination of visual and contact chemosensory inputs can induce persistent courtship in males. Additional studies have shown that moving [6] or immobile [7] dummies can induce male courtship if the putative courtship decision-making P1 neurons in the lateral protocerebrum (LPR) are simultaneously stimulated. We previously established a treadmill-based courtship assay, in which a stationary male anchored to a metal wire can walk on a freely moving Styrofoam ball [8] . Using this system, we demonstrated that the tethered male initiates courtship in response to a moving female abdomen, provided the male foreleg has come into contact with female pheromones by tapping a female body. We additionally showed that P1 neurons respond to female pheromones and, to a lesser extent, male pheromones [8] . However, it remains to be clarified how visual inputs impact the activities of P1 neurons. This study attempts to quantitatively analyse the contribution of vision to courtship control using a newly developed virtual reality technique in which moving light spots presented on a computer screen represent the courtship target for a male fly. We show that horizontal movement of a light spot initiates and maintains courtship-like following pursuit in wild-type males in the absence of female pheromone cues, provided that the fly is primed by optogenetic stimulation of either of two doublesex(dsx) -expressing neuronal clusters in the LPR, pC1 (P1) and pC2l. In contrast, males that are mutant for fruitless ( fru ), a key gene for sexual development of the nervous system [9] , do not require optogenetic priming of pC1 or pC2l to initiate courtship-like following pursuit in response to a moving light stimulus, particularly when they are group-reared as opposed to maintained in isolation for several days after eclosion. We further demonstrate that LPR neurons in group-reared fru mutant males exhibit enhanced responsiveness to visual stimuli as compared with wild-type or isolation-reared fru mutant males. Overall, our data indicate that enhanced responsiveness of LPR neurons to visual stimuli, as observed in fru mutants or as artificially imposed by optogenetic activation in wild-type males, mediates the motion-induced courtship-like pursuit even in the absence of chemosensory cues. Males initiate courtship-like pursuit toward moving light spots Previously, we showed that a male fly tethered to a metal wire displays quasi-normal courtship behaviour while walking on a treadmill upon tapping the female abdomen with his foreleg [8] . This observation was confirmed in the present study ( Fig. 1a ). After touching the female abdomen, the tethered male readily commences the courtship-like pursuit of this target, extending and vibrating a wing to generate courtship songs [8] . The courtship bouts typically cease within 1 min [8] . However, if a moving female abdomen is presented in front of the male, then the tethered male will exhibit sustained courtship-like pursuit until the target female stops ‘moving’ [8] . These results indicate that the courtship-like pursuit is visually guided [4] , [8] . In the present experiments, we found that a tethered male displayed sustained courtship-like pursuit even when the target female was replaced with a moving square-shaped light spot displayed on a screen ( Fig. 1b ), provided that he had tapped the female abdomen at least one time. We reasoned that the chemosensory stimuli offered to the male by tapping increased the excitability of certain neurons critical for initiating courtship, so that subsequent visual input could induce a sustained courtship-like pursuit. We therefore attempted to replace the chemosensory stimuli for courtship induction with optogenetic stimulation of neurons via channelrhodopsin-wide receiver (ChRWR), which can be activated by blue light irradiation [10] . Indeed, courtship-like pursuit was induced in a male without tapping when dsx -expressing neurons were stimulated via ChRWR while a moving light spot was being presented in front of him; the male ran to follow the target and extended/vibrated a wing to sing, while gradually turning his body axis (shown as Δ x ) according to the target position ( Fig. 1b–d ). Note that ChRWR-mediated stimulation by itself did not induce courtship-like pursuit in the male, nor did presentation of the moving light spot alone ( Supplementary Fig. 1 ). Previous studies have demonstrated that a dummy magnet is sufficient to initiate courtship pursuit by freely walking males [5] . It is possible that tethering the males, as was done in the present study, reduced their overall arousal level so that visual stimulation alone was unable to induce courtship-like pursuit. 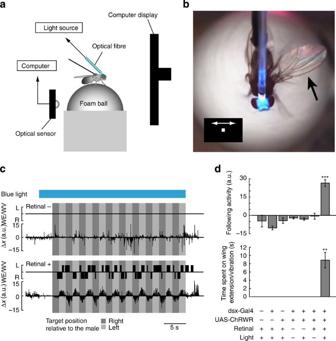Figure 1: Virtual reality paradigm for studyingDrosophilacourtship. (a) Experimental setup. A male fly is anchored by a metal wire on his dorsal thorax and allowed to walk on a Styrofoam ball, the movement of which is automatically monitored by an optical sensor connected to a computer. ChRWR activation is restricted to the brain by using an optic fibre to guide a light stimulus to the head. Visual stimuli are presented on a computer display. (b) An example of unilateral wing extension/vibration (arrow) of a tethered male on the treadmill induced by a moving square of light (inset) presented on a screen. (c) Ethogram for wing extension/vibration (WE/WV) and locomotion (Δx) in arbitrary units (a.u.) induced by a small square of light moving horizontally on the right (indicated by a dark grey background) or left (light grey background) side of the fly, which was fed a diet without (retinal−: control) or with (retinal+: test) retinal, which is essential for ChRWR activation. In the WE/WV records, a vertical bar represents the time at which a left (L) or right (R) wing opened (the anterior margin of the wing came to a position of 45° relative to the body axis). Δxrepresents the amount of displacement to the left or right direction for every 20 ms. Blue light to activate ChRWR was applied for the period shown above the motion records. (d) Following (upper graph) and WE/WV (lower graph) activities of the flies carryingdsx-Gal4and/orUAS-ChRWRwith or without retinal supplementation and light stimulation. The means±s.e.m. are shown. **P<0.01, ***P<0.001, Student’st-test. Test flies were compared with wild-type control flies that were fed retinal and subjected to light illumination. For both the following activity and wing extension/vibration, the numbers of flies in each group were 8, 11, 11, 8, 8, 8 and 8, respectively (in order from left to right). Figure 1: Virtual reality paradigm for studying Drosophila courtship. ( a ) Experimental setup. A male fly is anchored by a metal wire on his dorsal thorax and allowed to walk on a Styrofoam ball, the movement of which is automatically monitored by an optical sensor connected to a computer. ChRWR activation is restricted to the brain by using an optic fibre to guide a light stimulus to the head. Visual stimuli are presented on a computer display. ( b ) An example of unilateral wing extension/vibration (arrow) of a tethered male on the treadmill induced by a moving square of light (inset) presented on a screen. ( c ) Ethogram for wing extension/vibration (WE/WV) and locomotion (Δ x ) in arbitrary units (a.u.) induced by a small square of light moving horizontally on the right (indicated by a dark grey background) or left (light grey background) side of the fly, which was fed a diet without (retinal−: control) or with (retinal+: test) retinal, which is essential for ChRWR activation. In the WE/WV records, a vertical bar represents the time at which a left (L) or right (R) wing opened (the anterior margin of the wing came to a position of 45° relative to the body axis). Δ x represents the amount of displacement to the left or right direction for every 20 ms. Blue light to activate ChRWR was applied for the period shown above the motion records. ( d ) Following (upper graph) and WE/WV (lower graph) activities of the flies carrying dsx-Gal4 and/or UAS-ChRWR with or without retinal supplementation and light stimulation. The means±s.e.m. are shown. ** P <0.01, *** P <0.001, Student’s t -test. Test flies were compared with wild-type control flies that were fed retinal and subjected to light illumination. For both the following activity and wing extension/vibration, the numbers of flies in each group were 8, 11, 11, 8, 8, 8 and 8, respectively (in order from left to right). Full size image We next examined the efficacy of various visual stimuli in an effort to find the optimal visual stimulus for inducing courtship-like following pursuit. We discovered that horizontally aligned light spots (multi-spots) that moved in the horizontal direction at a high angular velocity (480° s −1 ) were twice as potent as a single moving spot (53° s −1 ) in inducing the courtship-like following pursuit when dsx -expressing neurons were simultaneously optogenetically activated ( Fig. 2a–c ). The maximal tracking responses were attained at temporal frequencies of 4–16 Hz ( Fig. 2d ) for stimuli consisting of square spots at 10–20° (viewing angle) in height ( Supplementary Fig. 2a ). The multi-spots were effective in inducing pursuit when presented in the centre of the visual field regardless of the direction of motion, whereas targets presented in the periphery of the visual field were only effective when they moved away from and not toward the centre of the visual field ( Supplementary Fig. 2b–d ). These results suggest that the test fly indeed turned in a direction so as to capture the moving targets at the centre of his visual field for tracking (that is, orienting movement). Similar to those males in which dsx -expressing neurons were primed via ChRWR-mediated stimulation as described above, males that were allowed to first tap a female also exhibited robust tracking activities in response to subsequent presentations of a moving spot or multi-spot stimulus without ChRWR-mediated neural stimulation ( Fig. 2e cf , Fig. 2c ). In fact, a single tap on a female was sufficient for maintaining the courtship-like following pursuit in the male for as long as 10 min, provided the moving multi-spot stimulus continued ( Supplementary Fig. 2e ). This observation raises the possibility that the sex-specific features of the target per se are not necessary to maintain the courtship-like following pursuit. To investigate this possibility, we performed an experiment in which the test male was allowed to tap either a female or male abdomen before the presentation of a moving female or male visual target. We found that the test male exhibited sustained pursuit of both male and female visual targets provided he had first tapped the female abdomen. On the other hand, test males that tapped the male abdomen did not initiate courtship-like pursuit of visual targets, even if the visual target was a female ( Fig. 2f ). These results are consistent with previous reports suggesting that inhibitory pheromones prevent males from courting inappropriate targets [11] , [12] . We conclude that once courtship is triggered, non-sex-specific moving targets, including artificial targets such as light spots, are sufficient for maintaining courtship-like following pursuit by males. 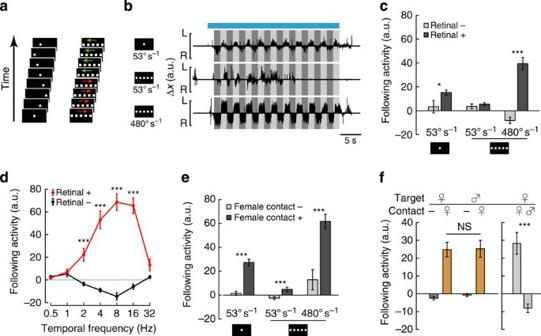Figure 2: Visually induced courtship-like pursuit after tapping or during ChRWR activation. (a) A single moving square of light (left-hand side) or a multi-spot pattern (right-hand side) was presented to a tethered fly. Each side of the light square corresponded to a visual angle of 15°. (b–d) ChRWR-mediated neuronal activation supersedes female tapping to elicit courtship-like following pursuit in a male. (b) Examples of locomotion records (Δx) of a fly in response to a single square of light (upper trace) or multi-spot pattern (middle and lower traces) moving at 53° s−1(upper and middle traces) or 480° s−1(lower trace) under illumination with blue light (shown above the ethogram). (c) Following activities in response to the moving squares of light as indicated in the bottom of the graph. *P<0.05, ***P<0.001, Student’st-test; the number of flies tested were 8, 9 and 8 for the bar, multi-spot (53° s−1) and multi-spot (480° s−1) stimuli under the retinal− conditions, and 6, 6 and 6 for these stimuli under the retinal+ conditions, respectively. (d) Following activity (ordinate) as a function of the temporal frequency (abscissa) of horizontal multi-spot pattern movement. ***P<0.001, Student’st-test;n=10 (retinal−) and 16 (retinal+). (e,f) Courtship induced by female tapping in the absence of ChRWR-mediated neuronal activation. (e) Following activity towards the visual patterns indicated on the bottom of the graph. ***P<0.001, Student’st-test; the numbers of flies tested were 22, 20 and 17 for the bar, multi-spot (53° s−1) and multi-spot (480° s−1) stimuli under the retinal− conditions, and 21, 17 and 17 for these stimuli under the retinal+ conditions, respectively. (f) Effects of the sex of the fly used as a visual target (target) and that used as a target for tapping (contact) on subsequent courtship-like pursuit (following activity). Means±s.e.m. are shown. NS, not significant; *P<0.05, **P<0.01, ***P<0.001, Student’st-test; the numbers of flies tested in each group were 18, 18, 16, 16, 10 and 8, respectively (in order from left to right). Figure 2: Visually induced courtship-like pursuit after tapping or during ChRWR activation. ( a ) A single moving square of light (left-hand side) or a multi-spot pattern (right-hand side) was presented to a tethered fly. Each side of the light square corresponded to a visual angle of 15°. ( b – d ) ChRWR-mediated neuronal activation supersedes female tapping to elicit courtship-like following pursuit in a male. ( b ) Examples of locomotion records (Δ x ) of a fly in response to a single square of light (upper trace) or multi-spot pattern (middle and lower traces) moving at 53° s −1 (upper and middle traces) or 480° s −1 (lower trace) under illumination with blue light (shown above the ethogram). ( c ) Following activities in response to the moving squares of light as indicated in the bottom of the graph. * P <0.05, *** P <0.001, Student’s t -test; the number of flies tested were 8, 9 and 8 for the bar, multi-spot (53° s −1 ) and multi-spot (480° s −1 ) stimuli under the retinal− conditions, and 6, 6 and 6 for these stimuli under the retinal+ conditions, respectively. ( d ) Following activity (ordinate) as a function of the temporal frequency (abscissa) of horizontal multi-spot pattern movement. *** P <0.001, Student’s t -test; n =10 (retinal−) and 16 (retinal+). ( e , f ) Courtship induced by female tapping in the absence of ChRWR-mediated neuronal activation. ( e ) Following activity towards the visual patterns indicated on the bottom of the graph. *** P <0.001, Student’s t -test; the numbers of flies tested were 22, 20 and 17 for the bar, multi-spot (53° s −1 ) and multi-spot (480° s −1 ) stimuli under the retinal− conditions, and 21, 17 and 17 for these stimuli under the retinal+ conditions, respectively. ( f ) Effects of the sex of the fly used as a visual target (target) and that used as a target for tapping (contact) on subsequent courtship-like pursuit (following activity). Means±s.e.m. are shown. NS, not significant; * P <0.05, ** P <0.01, *** P <0.001, Student’s t -test; the numbers of flies tested in each group were 18, 18, 16, 16, 10 and 8, respectively (in order from left to right). Full size image pC1 and pC2l neurons trigger male courtship To determine which subset of dsx -expressing neurons mediates the observed priming of visually guided courtship pursuit in males, we performed a behavioural Mosaic Analysis with Repressible Cell Marker (MARCM) analysis. We generated 73 males carrying ChRWR-expressing MARCM clones. Following the completion of behavioural assays with the virtual reality courtship paradigm, these flies were killed for histochemical identification of manipulated neurons that were selectively labelled by Venus fused to ChRWR ( Fig. 3a–d ). Among the dsx -expressing neuron clusters [13] , [14] stimulated via ChRWR, only the activation of pC1 and pC2l clusters was significantly correlated with the occurrence of both following and wing extension/vibration behaviours in courtship-like following pursuit of a multi-spot pattern ( Fig. 3e ). Furthermore, the pC2l cluster was also significantly correlated with the occurrence of proboscis extension and abdominal bending under similar conditions ( Fig. 3e ). In the later stages of natural courtship, the male fly licks the female genitalia by extending his proboscis and bends his abdomen in attempted copulation [15] , [16] . The pC1 cluster includes a male-specific fru -positive subset of cells (~20 cells), called the P1 cluster that has been shown to function as the decision-making centre for male courtship [8] , [17] , [18] . pC2l represents a non- fru -expressing sexually dimorphic cluster composed of ~35 cells [13] , [14] , [19] . By examining male flies with different patterns of ChRWR expression in pC1 and pC2l clusters, the functional differences in the contribution of these two neuron groups to courtship-like behaviour were revealed ( Fig. 3f and Supplementary Movies 1 , 2 ). First, male flies with either ChRWR-positive pC1 or pC2l clones exhibited pursuit of targets. In contrast, male flies that were ChRWR-negative in both pC1 and pC2l clones exhibited avoidance behaviour, as evidenced by the fact that they turned in the direction opposite to the target movement ( Fig. 3f ). Second, ChRWR-mediated stimulation of pC1 induced wing extension/vibration regardless of the direction of movement (left versus right) of the target in the visual field, whereas stimulation of pC2l induced wing extension/vibration only when the visual target moved in the direction opposite the hemisphere in which the pC2l clone was located. Thus, it appears that pC2l cluster neurons activate contralateral motor programmes, whereas pC1 neurons activate both contralateral and ipsilateral motor programmes for courtship-like wing extension/vibration that results in song generation. We speculate that while the pC1/P1 cluster neurons drive pC2l cluster neurons bilaterally, the pC2l cluster neurons rectify the pC1/P1-derived inputs so as to activate song motor programmes only on the side closer to the target, ensuring the appropriately directed unilateral wing extension/vibration by the courting male. The pC2l cluster neurons exhibited similar direction-selectivity in both proboscis extension and abdominal bending as in wing extension/vibration ( Fig. 3f ). In contrast, neither pC1 nor pC2l cluster neurons exhibited direction-selectivity in inducing target tracking, despite the fact that tracking involves a lateralized component, that is, turning to the left or right. When a stronger blue light stimulus was used (~280% increase in intensity), ChRWR-mediated stimulation of pC1 or pC2l cluster neurons alone induced locomotion and wing extension/vibration and, in addition, proboscis extension and abdominal bending in the case of pC2l activation, even in the absence of visual stimulations ( Supplementary Fig. 3 ). These results suggest that pC1 cluster neurons release motor programmes for the early phase of courtship, while pC2l cluster neurons release both the early- and late-phase programme, that is, licking and attempted copulation. 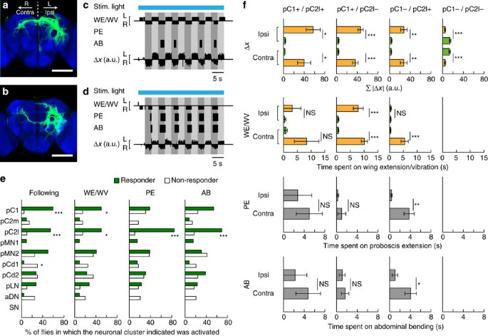Figure 3: Identification of neurons involved in visually induced courtship. (a–d) Examples of pC1- (a) and pC2l- (b) cluster MARCM clones expressing ChRWR::Venus in two flies that yielded the ethograms shown incandd, respectively. Shown are the frontal views of the brain, the laterality of which is indicated by the arrows (R, the right hemisphere; L, the left hemisphere; Contra, the side contralateral to the somata; Ipsi, ipsilateral to the somata). Both ethograms include WE/WV, proboscis extension (PE), abdominal bending (AB) and Δx. Scale bar, 100 μm. (e) Proportions of flies with ChRWR-positive mosaic clones in a givendsx-expressing cluster for responders (flies that displayed a given courtship element; filled bars) or non-responders (flies that did not display a given courtship element; open bars). The courtship elements and the names of the clusters analysed are indicated above and on the left-hand side of each graph, respectively. The significance of the differences was evaluated by Fisher’s exact probability test for each neural cluster on 2 × 2 matrices. *P<0.05, ***P<0.001,n=73. (f) Quantification of four courtship elements (Δx, WE/WV, PE and AB) in flies carrying ChRWR::Venus-positive MARCM clones in both pC1 and pC2l (pC1+/pC2l+), either of them (pC1+/pC2l− and pC1−/pC2l+) or neither of them (pC1−/pC2l−). Data were classified on the basis of two criteria: (i) whether the behavior was induced by the visual pattern movement toward (ipsi) or by that away from (contra) the side in which the somata of neurons of concern were situated and (ii) whether the behavior was induced in/toward the same side as (yellow) or the side opposite to (green) the direction of stimulus movement. Criterion (i) could not be applied to pC1−/pC2l− flies, and thus the relationship between the directions of fly movement and those of the visual stimulus was used to categorize the data instead. NS, not significant; *P<0.05, ***P<0.01, ***P<0.001 by the pairedt-test (Δx) or the Wilcoxon signed rank test (WE/WV, PE and AB).n=4, 15, 19 and 38 for pC1+/pC2l+, pC1+/pC2l−, pC1−/pC2l+ and pC1−/pC2l−, respectively. Means±s.e.m. are shown. Figure 3: Identification of neurons involved in visually induced courtship. ( a – d ) Examples of pC1- ( a ) and pC2l- ( b ) cluster MARCM clones expressing ChRWR::Venus in two flies that yielded the ethograms shown in c and d , respectively. Shown are the frontal views of the brain, the laterality of which is indicated by the arrows (R, the right hemisphere; L, the left hemisphere; Contra, the side contralateral to the somata; Ipsi, ipsilateral to the somata). Both ethograms include WE/WV, proboscis extension (PE), abdominal bending (AB) and Δ x . Scale bar, 100 μm. ( e ) Proportions of flies with ChRWR-positive mosaic clones in a given dsx -expressing cluster for responders (flies that displayed a given courtship element; filled bars) or non-responders (flies that did not display a given courtship element; open bars). The courtship elements and the names of the clusters analysed are indicated above and on the left-hand side of each graph, respectively. The significance of the differences was evaluated by Fisher’s exact probability test for each neural cluster on 2 × 2 matrices. * P <0.05, *** P <0.001, n =73. ( f ) Quantification of four courtship elements (Δ x , WE/WV, PE and AB) in flies carrying ChRWR::Venus-positive MARCM clones in both pC1 and pC2l (pC1+/pC2l+), either of them (pC1+/pC2l− and pC1−/pC2l+) or neither of them (pC1−/pC2l−). Data were classified on the basis of two criteria: (i) whether the behavior was induced by the visual pattern movement toward (ipsi) or by that away from (contra) the side in which the somata of neurons of concern were situated and (ii) whether the behavior was induced in/toward the same side as (yellow) or the side opposite to (green) the direction of stimulus movement. Criterion (i) could not be applied to pC1−/pC2l− flies, and thus the relationship between the directions of fly movement and those of the visual stimulus was used to categorize the data instead. NS, not significant; * P <0.05, *** P <0.01, *** P <0.001 by the paired t -test (Δ x ) or the Wilcoxon signed rank test (WE/WV, PE and AB). n =4, 15, 19 and 38 for pC1+/pC2l+, pC1+/pC2l−, pC1−/pC2l+ and pC1−/pC2l−, respectively. Means±s.e.m. are shown. Full size image Neural activities that correlate with courtship A previous Ca 2+ imaging study [8] demonstrated that the pC1/P1 cluster neurons are activated by female sex pheromones, which stimulate foreleg sensory cells when the male taps the female abdomen [20] . To determine whether the pC1 and pC2l cluster neurons are also active during subsequent courtship bouts maintained by visual stimuli, that is, the presentation of a moving multi-spot pattern, we imaged activity in tethered male flies expressing GCaMP3.0 in dsx-Gal4 positive neurons while they engaged in courtship-like following behaviour on the treadmill ( Fig. 4a–c , Supplementary Movie 3 ). The dsx- positive neurons in the LPR exhibited a discrete Ca 2+ rise upon tapping of the female abdomen ( Fig. 4a–c,e and Supplementary Fig. 4a ). Subsequent presentations of the multi-spot visual target elicited similar Ca 2+ rises ( Fig. 4e and Supplementary Movie 3 ). Next, we performed similar experiments in male flies harbouring GCaMP3.0-expressing MARCM clones. In response to the multi-spot pattern, the pC1 and pC2l cluster neurons displayed periodic Ca 2+ increases that coincided with turns of the fly toward the hemisphere in which the clones were located ( Fig. 4f–i and Supplementary Fig. 4b,c ). To our knowledge, this is the first study to capture neural correlates of the courtship-like pursuit maintenance in Drosophila . 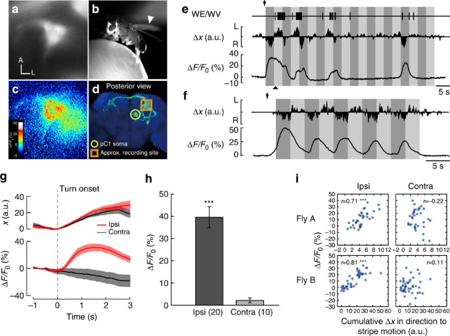Figure 4: Neural correlates of courtship. (a) Raw fluorescent image capturing GCaMP3.0 expression in the LPR. (b) The male displayed unilateral wing vibration (arrowhead) during Ca2+imaging. (c) Pseudocolour image of fluorescent change in neurons upon female tapping (indicated by arrowhead ine). (d) pC1 clone yielded the Ca2+activity recordings shown inf. (e) Ca2+activity changes (ΔF/F0, %) in the LPR in response to female tapping (indicated by a vertical arrow at the top of the panel) and the subsequent multi-spot stimulus (direction of movement indicated by background colour: dark grey, right; light grey, left) are shown with an ethogram. (f) Ca2+responses from the MARCM clone neurons during male courtship in the virtual reality paradigm. A male fly carrying the pC1 clone in the right hemisphere exhibited courtship-like pursuit (top trace) and periodic Ca2+increases in the pC1 clone (bottom trace) in response to female tapping and the subsequent multi-spot stimulus. (g) Average locomotion and Ca2+responses synchronized by the onset of body turning to the direction relative to the neuronal somata (ipsilateral versus contralateral) for pC1. A total of 20 ipsilateral turns and 10 contralateral turns were observed in four male flies. Shaded region represents range defined by the s.e.m. (h) Quantitative comparisons of Ca2+-response amplitude between events associated with ipsilateral turns and those associated with contralateral turns in pC1. The maximal ΔF/F0values in the initial 3 s after the onset of turning were averaged. The number below the graph represents the number of turns used to calculate the average response amplitude.n=4 flies. Means±s.e.m. are shown. (i) Scatter plots for Ca2+response amplitude in pC1 as a function of cumulative locomotion activity, Δx. Pearson’s correlation coefficient (r) indicates that Ca2+changes coincided with ipsilateral but not contralateral turns. ThePvalues and 95% confidence intervals for the correlation coefficients are as follows: Fly A (ipsi):P<0.001, 0.49–0.84; Fly A (contra):P>0.05, −0.52–0.12; Fly B (ipsi):P<0.001, 0.68–0.89; Fly B (contra):P>0.05, −0.19–0.38. ***P<0.001. The number of analysed data points was 35 and 45 for Fly A and B, respectively. Figure 4: Neural correlates of courtship. ( a ) Raw fluorescent image capturing GCaMP3.0 expression in the LPR. ( b ) The male displayed unilateral wing vibration (arrowhead) during Ca 2+ imaging. ( c ) Pseudocolour image of fluorescent change in neurons upon female tapping (indicated by arrowhead in e ). ( d ) pC1 clone yielded the Ca 2+ activity recordings shown in f . ( e ) Ca 2+ activity changes (Δ F / F 0 , %) in the LPR in response to female tapping (indicated by a vertical arrow at the top of the panel) and the subsequent multi-spot stimulus (direction of movement indicated by background colour: dark grey, right; light grey, left) are shown with an ethogram. ( f ) Ca 2+ responses from the MARCM clone neurons during male courtship in the virtual reality paradigm. A male fly carrying the pC1 clone in the right hemisphere exhibited courtship-like pursuit (top trace) and periodic Ca 2+ increases in the pC1 clone (bottom trace) in response to female tapping and the subsequent multi-spot stimulus. ( g ) Average locomotion and Ca 2+ responses synchronized by the onset of body turning to the direction relative to the neuronal somata (ipsilateral versus contralateral) for pC1. A total of 20 ipsilateral turns and 10 contralateral turns were observed in four male flies. Shaded region represents range defined by the s.e.m. ( h ) Quantitative comparisons of Ca 2+ -response amplitude between events associated with ipsilateral turns and those associated with contralateral turns in pC1. The maximal Δ F / F 0 values in the initial 3 s after the onset of turning were averaged. The number below the graph represents the number of turns used to calculate the average response amplitude. n =4 flies. Means±s.e.m. are shown. ( i ) Scatter plots for Ca 2+ response amplitude in pC1 as a function of cumulative locomotion activity, Δ x . Pearson’s correlation coefficient ( r ) indicates that Ca 2+ changes coincided with ipsilateral but not contralateral turns. The P values and 95% confidence intervals for the correlation coefficients are as follows: Fly A (ipsi): P <0.001, 0.49–0.84; Fly A (contra): P >0.05, −0.52–0.12; Fly B (ipsi): P <0.001, 0.68–0.89; Fly B (contra): P >0.05, −0.19–0.38. *** P <0.001. The number of analysed data points was 35 and 45 for Fly A and B, respectively. Full size image Socialization urges neurons to trigger courtship As shown in Fig. 2e , wild-type males initiated courtship pursuit on tapping the female. Under tethered conditions, wild-type males only initiated courtship-like pursuit if they first tapped a female abdomen ( Fig. 5a ); courtship-like pursuit was not initiated by tapping a male abdomen [8] ( Fig. 2f ). In contrast to wild-type males, male-to-male courtship is prevalent among fru mutant males [21] . We therefore analysed the courtship behaviour of fru sat homozygous males using our virtual reality behavioural assay. Strikingly, fru sat males initiated courtship toward a moving multi-spot stimulus without prior tapping ( Fig. 5a and Supplementary Movies 4 , 5 ), suggesting that fru sat mutant males do not require priming for courtship by pheromone sensation via tapping. Rather, fru sat males were hypersensitive to visual stimuli and readily initiated courtship-like pursuit without prior chemosensory cues. 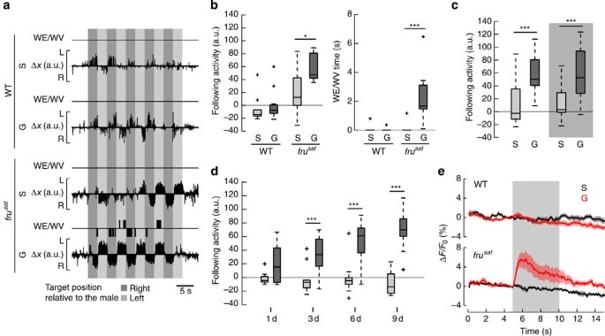Figure 5: Neural correlates of experience-dependent courtship-like following pursuit infrumutant males. (a,b) Courtship-like activity toward horizontal movements of the multi-spot pattern in wild-type (CS) andfrumutant males. Males were presented visual patterns without a prior female tapping. (a) Representative behaviour records in the wild-type (WT; upper two panels) andfrumutant (lower two panels). The files were reared singly (S) or in a group (10 flies per vial; G) for 6 days. (b) Quantified following activities (left) and wing displays (right) in wild-type andfrumutant reared in isolation (S) or groups (G).n=12 (wild type, S and G), 8 (frumutant, S) and 7 (frumutant, G) flies. (c) Quantified following activities of group- (G) and isolation- (S) rearedfrusatmales kept under a 12:12 light–dark cycle (white background,n=12 for each of S and G) or constant darkness (shaded background,n=13 and 10 for S and G, respectively) for 6–9 days. (d) Ontogeny of visually induced courtship-like pursuit.frusatmale flies were group-reared (filled boxes) or kept in isolation (open boxes) for 1, 3, 6 or 9 days after eclosion. The numbers of flies tested 1, 3, 6 or 9 days after eclosion were 12, 10, 10 and 9 (single-reared) and 12, 10, 9 and 9 (group-reared), respectively. (e) Average Ca2+responses recorded from the ipsilateral LPR upon stimulation with moving multi-spot patterns in wild-type (upper panel) orfrumutant males (lower panel) that were group-reared (G) or those reared in isolation (S);n=5 flies tested for group-reared or single-reared wild-type and single-rearedfrumutant males, andn=10 for group-rearedfrumutant males. Traces represent the mean optical responses, and the s.e.m. is indicated by the areas coloured in pale red and black for grouped and isolated flies, respectively. Shading on background indicates stimulus period. Upper/lower limit and inner horizontal lines of the box plots represent upper/lower quartile and median, respectively; whiskers indicate 1.5 × interquartile range from upper/lower quartiles. Values beyond whiskers are indicated by ‘+’. *P<0.05, ***P<0.001, Mann–Whitney’sU-test. Figure 5: Neural correlates of experience-dependent courtship-like following pursuit in fru mutant males. ( a , b ) Courtship-like activity toward horizontal movements of the multi-spot pattern in wild-type (CS) and fru mutant males. Males were presented visual patterns without a prior female tapping. ( a ) Representative behaviour records in the wild-type (WT; upper two panels) and fru mutant (lower two panels). The files were reared singly (S) or in a group (10 flies per vial; G) for 6 days. ( b ) Quantified following activities (left) and wing displays (right) in wild-type and fru mutant reared in isolation (S) or groups (G). n =12 (wild type, S and G), 8 ( fru mutant, S) and 7 ( fru mutant, G) flies. ( c ) Quantified following activities of group- (G) and isolation- (S) reared fru sat males kept under a 12:12 light–dark cycle (white background, n =12 for each of S and G) or constant darkness (shaded background, n =13 and 10 for S and G, respectively) for 6–9 days. ( d ) Ontogeny of visually induced courtship-like pursuit. fru sat male flies were group-reared (filled boxes) or kept in isolation (open boxes) for 1, 3, 6 or 9 days after eclosion. The numbers of flies tested 1, 3, 6 or 9 days after eclosion were 12, 10, 10 and 9 (single-reared) and 12, 10, 9 and 9 (group-reared), respectively. ( e ) Average Ca 2+ responses recorded from the ipsilateral LPR upon stimulation with moving multi-spot patterns in wild-type (upper panel) or fru mutant males (lower panel) that were group-reared (G) or those reared in isolation (S); n =5 flies tested for group-reared or single-reared wild-type and single-reared fru mutant males, and n =10 for group-reared fru mutant males. Traces represent the mean optical responses, and the s.e.m. is indicated by the areas coloured in pale red and black for grouped and isolated flies, respectively. Shading on background indicates stimulus period. Upper/lower limit and inner horizontal lines of the box plots represent upper/lower quartile and median, respectively; whiskers indicate 1.5 × interquartile range from upper/lower quartiles. Values beyond whiskers are indicated by ‘+’. * P <0.05, *** P <0.001, Mann–Whitney’s U -test. Full size image It is known that fru mutant males, when placed together, will form a chain of suitors such that a male will court another male while being courted by yet another male [21] . The chaining behaviour is exaggerated if mutant males are reared together for several days [22] . Thus, the tendency to engage in homosexual courtship appears to be socially modulated. We suspected that the enhanced chaining in group-reared fru sat males might result from the elevated responsiveness of these flies to visual stimuli. Indeed, fru sat males initiated courtship-like pursuit in response to multi-spot patterns at significantly higher rates after being reared in a group for 3–9 days, as compared with the rate estimated on the day of eclosion ( Fig. 5a–d ). On the other hand, fru sat males reared in isolation for an extended period (up to 9 days) did not exhibit visually induced courtship-like pursuit ( Fig. 5d ) in the manner of the group-reared fru sat males, suggesting that the fru sat males were primed for courtship-like behaviour by social interactions rather than by aging. The visual hypersensitivity exhibited by group-reared fru sat males did not depend on early visual experience, as evidenced by the observation that group rearing resulted in an increase in courtship-like pursuit even when fru sat males were maintained in darkness between eclosion and testing ( Fig. 5c ). We additionally examined whether the responsiveness of LPR neurons to visual pattern stimuli is increased by group rearing in fru sat males. As shown in Fig. 5e , LPR neurons in group-reared fru sat males exhibited robust Ca 2+ rises upon visual pattern stimulation, whereas LPR neurons in isolation-reared fru sat males did not ( Fig. 5e ). It is an intriguing possibility that the elevated visual responsiveness of LPR neurons may be responsible for the increase in visually induced courtship-like pursuit in fru sat males. For quantitative analysis of male courtship behaviour, this study established a virtual reality paradigm in which moving light spots displayed on a computer screen acted as virtual courtship targets for tethered male flies. By combining MARCM techniques, Ca 2+ imaging and optogenetic stimulation of LPR neurons with the virtual reality paradigm, we demonstrated that two dsx -expressing clusters in the LPR, pC1 and pC2l, have key roles in inducing courtship-like behaviour: optogenetic activation of either pC1 or pC2l led to initiation of courtship-like behaviour in males viewing moving light spots. Moreover, both pC1 and pC2l clusters exhibited periodic Ca 2+ rises that coincided in time with left or right turns of the courting male fly. Although both clusters similarly drove courtship-like pursuit, pC1 stimulation resulted in unilateral wing extension and vibration on both sides, whereas pC2l stimulation resulted in wing displays only on the side contralateral to the cluster. In addition, pC2l but not pC1 activation induced abdominal bending and proboscis extension. Thus, while the functions of pC1 and pC2l overlap in driving courtship-like pursuit, they appear to serve distinct functional roles in other aspects of courtship-like behaviour. Although our artificial activation experiments demonstrated the sufficiency of pC1 and pC2l clusters in inducing aspects of courtship-like behaviour, the necessity of these neural clusters for the induction of courtship-like behaviour was not examined due to the technical difficulties inherent to the stochastic nature of MARCM clone production, that is, bilateral clones of a given cluster were rarely obtained. Our results further suggest that fru mutant males are hypersensitive to visual stimuli, as they initiated courtship-like pursuit in response to moving multi-spot patterns without prior chemosensory priming, that is, tapping of the target ( Fig. 5a ). Interestingly, visually induced courtship-like following behaviour was enhanced by group rearing of fru mutant males. It is conceivable that fru mutant males rely on visual cues with lower target specificity, resulting in nondiscriminatory sex-independent courtship. We were able to visually induce courtship-like behaviour in wild-type males, similar to that seen in fru mutant males, by first optogenetically activating dsx -expressing neurons ( Fig. 2b,c ). We speculate that the visual responsiveness of courtship triggering neurons of fru sat males is enhanced, resulting in the initiation of courtship-like behaviour by inappropriate visual targets. In support of this claim, we observed that moving multi-spot stimuli evoked robust Ca 2+ responses in LPR neurons in fru mutant males that were group-reared but not in those kept in isolation ( Fig. 5e ). These results constitute the first observation of social experience-dependent changes in neural activities induced by a behaviour-relevant stimulus during courtship performance in Drosophila . Inagaki et al . [23] reported that group rearing of wild-type males resulted in an elevated threshold for initiating courtship upon stimulation of P1 (a subset of pC1) cluster neurons with a red-shifted channelrhodopsin (ReaChR), and that P1 cluster neurons generated smaller Ca 2+ responses upon ReaChR activation in group-reared males as compared with isolation-reared males. Thus, it appears that group rearing reduces pC1/P1 neuron excitability in the wild-type males and increases it in the fru sat males. Although it remains to be clarified why group rearing exerts these contrasting effects on wild-type and fru mutant males, the pC1 cluster neurons are obvious candidates for substrates where the excitatory state is modulated for appropriate courtship performance by social experience. The present findings thus open an avenue for unravelling the mechanisms by which experience shapes behaviour at the level of single identified neurons. Fly strains Flies were reared on a cornmeal–yeast medium under a 12/12 h light–dark cycle at 25 °C. The dsx-Gal4 was a gift from S. Goodwin. fru sat was generated in our laboratory [24] . Other fly stocks except for UAS-ChRWR::Venus were obtained from the Bloomington Stock Center. To generate UAS-ChRWR::Venus transgenic flies, the pVenus-N1-ChRWR plasmid was obtained from H. Wang and H. Yawo [10] . The DNA fragment containing ChRWR::Venus was excised with the EcoR I and Not I restriction enzymes, then introduced to EcoR I-Not I restriction sites of the pUAST vector. With this construct, the UAS-ChRWR::Venus strain was established by P-element-mediated transformation using the w 1118 strain as a host. The genotype of flies used for optogenetic activation of dsx -expressing neurons ( Figs 1 and 2 ) was w 1118 ; dsx-Gal4 / UAS-ChRWR and that for Ca 2+ imaging ( Fig. 4 ) was w 1118 ; dsx-Gal4 , UAS-GCaMP3.0 / UAS-GCaMP3.0 . The flies of y hs-flp ; FRTG13 tubP-Gal80 / FRT G13; dsx-Gal4 / UAS-ChRWR::Venus genotype were used to generate mosaic clones of dsx -neurons expressing ChRWR ( Fig. 3 ) and the flies of y hs-flp ; FRTG13 tubP-Gal80 / FRT G13 ; dsx-Gal4 , UAS-GCaMP3.0/UAS-GCaMP3.0 genotype were used to generate mosaic clones of dsx -neurons expressing GCaMP3.0 ( Fig. 4 ). The genotypes of flies used in the behavioural experiment and Ca 2+ imaging experiment in Fig. 5 were Canton-S (wild type), w 1118 ; fru sat ( fru mutant), w 1118 ; dsx-Gal4 , UAS-GCaMP3.0 /+ (wild type) and w 1118 ; fru sat , dsx-Gal4 / fru sat , UAS-GCaMP3.0 ( fru mutant). Locomotion simulator In principle, the locomotion simulator was the same as described in previous studies [8] , [25] . According to the procedure described in the next section, a subject fly was tethered with a metal wire on its dorsal thorax and positioned over an air-supported Styrofoam ball of 6 mm in diameter. The fly could easily rotate the floating ball using just its legs, and could thus ‘walk’ and remain in a stationary position due to the tether. Locomotion of the fly was recorded by monitoring the rotations of the Styrofoam ball using an optical computer mouse sensor (ADNS2620; AVAGO Technologies). The sensor detected surface texture changes due to movements of the ball in the horizontal (Δ x ) and vertical (Δ y ) direction, in proportion to the ball’s rotation along the yaw and pitch axis, respectively. The Δ x and Δ y values, together with timestamps, were sent to a computer at 50 Hz via an Arduino Uno microcontroller with a custom sketch programme, then stored on a hard disk of the computer. When necessary, fly behaviour was video-recorded from above and/or from the left side of the fly at 29.97 or 30 frames per second (f.p.s. ), in addition to the recording of locomotion as described above. A custom programme written in LabView (National Instruments) generated the trigger signals for presenting visual patterns, for the delivery of excitation light for ChRWR, for recording locomotion and for video-monitoring of other types of behaviour, via a digital–analogue interface (USB-6259; National Instruments), RS-232C port and USB port. Fly rearing after eclosion Flies were collected within 4 h after eclosion and kept singly or in groups in a plastic vial with cornmeal–yeast medium. The inner dimensions of the vial were 14 mm and ~60 mm in diameter and length, respectively. Every 2–3 days, the flies were transferred to new vials with fresh medium until the day of the experiments to keep them clean. The flies used in the experiments that involved fru mutants were reared with extra care by inserting a small piece of wet Kimwipe onto the medium for humidification and to provide a foothold for the flies. For single and group rearing, 1 and 10 males of the same genotype were kept in one vial, respectively. Fly preparation for behaviour analysis Under cold anaesthesia, a short copper wire of ~150 μm in diameter and 3 mm in length was attached to the dorsal thorax of each male using ultraviolet glue. Then the males were kept singly in individual plastic chambers of 35 mm in diameter and 10 mm in height, which were humidified by a piece of wet filter paper placed on the floor. After allowing an ~2 h rest in the chamber, the free end of the copper wire (the end that was not affixed to the thorax) was attached to the fly holder, and then the fly was carefully positioned over an air-supported Styrofoam ball on the locomotion simulator so that the ball rotated smoothly along with the locomotion of the fly. Optogenetic activation of dsx -expressing neurons Optogenetic activation of neurons was carried out on flies that were collected ~8 h after eclosion and kept in a vial with the food medium for 3–5 days. At 2–3 days before their use in the experiments, the flies were transferred to a new vial with the retinal-containing food medium; an aliquot of all- trans retinal (R2500; Sigma) at 50 mg ml −1 in 100% ethanol was dropped on the food medium so as to form a uniform layer of 0.3 mg cm −2 on the medium surface. To avoid the possible activation of dsx -expressing neurons by environmental light, the flies fed retinal were kept in the dark until they were used in the experiments. The control fly groups were handled as the experimental groups were, except that they were transferred to a new vial containing the food medium without retinal 2–3 days before use. Light stimulation of brain neurons in a tethered male Excitation light to activate ChRWR was delivered to a fly on the locomotion simulator through a custom-made optical fibre cannula (diameter: 200 μm; NA: 0.39; Thorlabs), which was optically coupled to an LED light source (M470F1; peak wavelength: 460 nm; output: 10.1 mW; Thorlabs). The light was focused on the dorsal head region delineated by the left and right compound eyes. The light on/off and lighting duration were controlled by electrical signals fed to the LED driver (LEDD1B; Thorlabs). Illuminating the head per se did not elicit obvious behaviour except for increased locomotion in some flies. Visual stimulus Visual stimuli were generated by custom python scripts using Vision Egg, an open-source library for visual stimulus generation [26] . The multi-spot visual stimulus was made with a horizontal square grating patterned at a spatial frequency of 30° or 60°. Some parts of the grating pattern were masked with black when the stimulus needed to be given to a limited area in the fly’s visual field. The visual pattern was moved horizontally at a speed of 15–960° s −1 , corresponding to a temporal frequency (speed/spatial frequency) of 0.25–32 Hz. All the visual patterns were morphed so that the view angles of visual objects were unchanged regardless of their position in the fly’s visual field. The computer-generated images were shown on a display (XL2420T; resolution: 1,920 × 1,080 pixels; BenQ) at a frame rate of 120 f.p.s., which was confirmed by video-recording the display at 500 f.p.s. using a high-speed camera. The display was placed 15 cm in front of the tethered fly, covering an area of the fly’s visual field corresponding to ~120° in width and 67° in height, yielding a spatial resolution of ~0.1°. Mosaic analysis To generate mosaic flies that express ChRWR::Venus or GCaMP3.0 in subsets of dsx -expressing neurons, eggs were collected at ~24 h after eclosion and heat-shocked at 37 °C for 45 min. After the behaviour/imaging experiment, the mosaic flies were killed for the histological identification of ChRWR::Venus -positive or GCaMP3.0 -positive neurons. Immunohistochemical staining was carried out by using the following antibodies at the indicated dilutions: mouse monoclonal nc82 (1:10), rabbit polyclonal anti-GFP (1:1,000; Molecular Probes), Alexa546-conjugated goat anti-mouse IgG (1:200; Invitrogen) and Alexa488-conjugated goat anti-rabbit IgG (1:200; Invitrogen). ChRWR::Venus and GCaMP3.0 were detected by the anti-GFP antibody because both Venus and GCaMP3.0 were derivatives of GFP. The stained brains were reconstituted as a series of optical sections with intervals of 1.5 μm using a confocal microscope (LSM510 META; Carl Zeiss). The acquired images were processed and examined using ImageJ [27] . Analysis of courtship behaviour Following activity was quantified by Δ x values of the tracking sensor output, which correspond to the magnitude of turns the fly made to the left and right directions. Following activity was defined as: ∑|Δ x ipsi |−∑|Δ x contra |, where Δ x ipsi and Δ x contra were deviations toward (ipsilateral to) and away from (contralateral to) the direction of target motion at each time point, respectively. Analysis of courtship behavioural acts In quantifying the wing motion, we defined the time that the wing was opened or closed as the time when the anterior margin of a wing came up or down at 45° relative to the fly’s midline, and these times were manually recorded. We used two landmark lines crossing at 45° to each other, which were overlaid on the video-recorded dorsal images of the fly to judge whether the wing opened or not. The overlaying of landmark lines and video annotation were controlled by a custom macro programme in ImageJ and Vcode [28] , respectively. The quantification of licking and abdominal bending was accomplished in a similar manner using video images taken from the left side of the fly. We judged that licking occurred when the proboscis was extended for a distance 1.3 times or more of its length at rest. We judged that abdominal bending occurred when the abdomen was sufficiently bent that an imaginary line connecting the haltere and the abdominal tip came to meet at an angle of 15° or more to the thoracic midline. Calcium imaging The subject fly was cold-anaesthetized and the head was immobilized by fixing it to the thorax with ultraviolet glue. Next, the fly was attached to a sample holder (similar to that described in Seelig et al . [29] ) at its dorsal thorax; the fly was positioned so that the dorsal portion of the head delineated by the left and right compound eyes was exposed to the outside through a window made on the sample holder. To allow observation of the LPR where the recordings were to be made, the upper side of the sample holder was bathed in saline and a portion of the head cuticle was cut and removed with the edge of a syringe. After removing some of the fat bodies, tracheae running on the dorsal brain surface were focally peeled off and put aside using fine forceps with great caution. Finally, the saline was removed and the opening on the head capsule was sealed with transparent silicone gel (KWIK-SIL; World Precision Instruments), through which the fluorescent images were acquired. For GCaMP3.0 excitation, a metal halide ramp (KMH-250; Kiyohara Optics) was used as a light source. An excitation filter BP 470/40 nm, dichroic mirror FT 495 nm and emission filter BP 525/50 nm were applied. The intensity of the excitation light was adjusted by ND filters so that the mean baseline intensity of GCaMP3.0 fluorescence exceeded 1,000 at around the LPR region. The application of excitation light for ChRWR may interfere with fly vision. To minimize this undesirable effect, the aperture of excitation light was set to be as small as possible while still allowing uniform illumination around the target brain region. Fluorescent images were captured with a CCD camera (C7780-10; Hamamatsu Photonics; bit depth: 12 bit) or CMOS camera (ORCA-Flash4.0; Hamamatsu Photonics; bit depth: 16 bit), which was controlled by Aquacosmos (Hamamatsu Photonics) or HCImage (Hamamatsu Photonics). The binning of the cameras was set to 8 × 8 or 4 × 4, which gives spatial resolution of 1.28 × 1.28 μm for C7780-10 and 0.63 × 0.63 μm for ORCA-Flash4.0, respectively. Using a × 40 water immersion objective lens (W Plan Apochromat; Carl Zeiss), fluorescent images of the dsx -expressing neurons in the LPR were acquired and recorded at a frame rate of 9.1 or 10 Hz. To stimulate the male foreleg with the female body, the abdomen of a virgin female was attached to a thin needle held by a manual micromanipulator, and brought into contact with the male’s foreleg with the aid of live video images captured by an IR camera. To visually stimulate the fly, visual patterns were shown on a computer display placed ~15 cm in front of the male. A small portion of the display was hid behind the optical table for imaging and the sample holder, and thus the visual patterns were presented outside of this hidden region, that is, in the range of ~120° and ~30° in the horizontal and vertical direction of the fly’s visual field, respectively. Bleed-through of the light from the display increased the baseline signal value in the acquired fluorescent images. However, its effect on measurement of the response dynamics was negligible because there was no significant change in the signals due to the bleed-through before and during the motion of the grating pattern. Image analysis To measure the Ca 2+ responses in the dsx -expressing neurons, two rectangular regions of interest (ROIs) 20 or 30 pixels on each side, one on the dsx -expressing neurons in the LPR and the other on a brain region without GCaMP3.0 expression, were chosen for measurements. For each frame, the average fluorescence intensity of pixels within each of the ROIs was calculated, and the value for the ROI without GCaMP3.0 was subtracted from the value for the other ROI to obtain a crude fluorescent intensity value derived from GCaMP3.0 . Next, the crude fluorescent intensity value was corrected for photobleaching by subtracting the baseline value. The baseline value was estimated by fitting, by a single exponential function, the crude fluorescent intensity value in frames before the stimulus onset and in frames ranging from 3 s after the end of visual stimulus to the end of the recording. The Ca 2+ response was calculated as a fractional fluorescence change (Δ F / F 0 ). F 0 was the average of 10 frames before the onset of female contact or visual stimulus. Δ F was obtained by subtracting F 0 from the fluorescent value at each time point. Then Δ F was divided by F 0 and multiplied by 100. For quantitative comparisons of the response, the average Δ F / F 0 values from five frames around the peak response in the time range of interest were used. All the image processing was done on ImageJ using custom macro programmes, and all the calculations were done with a custom python script except for baseline fitting, which was performed on Igor Pro version 6.22J (Wave Metrics). How to cite this article: Kohatsu, S. et al . Visually induced initiation of Drosophila innate courtship-like following pursuit is mediated by central excitatory state. Nat. Commun , 6:6457 doi: 10.1038/ncomms7457 (2015).